Kv3.1 uses a timely resurgent K+current to secure action potential repolarization High-frequency action potential (AP) transmission is essential for rapid information processing in the central nervous system. Voltage-dependent K v 3 channels play an important role in this process thanks to their high activation threshold and fast closure kinetics, which reduce the neuron’s refractory period. However, premature K v 3 channel closure leads to incomplete membrane repolarization, preventing sustainable AP propagation. Here, we demonstrate that K v 3.1b channels solve this problem by producing resurgent K + currents during repolarization, thus ensuring enough repolarizing power to terminate each AP. Unlike previously described resurgent Na + and K + currents, K v 3.1b’s resurgent current does not originate from recovery of channel block or inactivation but results from a unique combination of steep voltage-dependent gating kinetics and ultra-fast voltage-sensor relaxation. These distinct properties are readily transferrable onto an orthologue K v channel by transplanting the voltage-sensor’s S3–S4 loop, providing molecular insights into the mechanism by which K v 3 channels contribute to high-frequency AP transmission. Voltage-gated potassium (K v ) channels create potassium-selective transmembrane pathways that alter their conducting state as a function of membrane potential. To this end, K v channels possess voltage-sensing domains (VSD) that detect changes in membrane potential and translate this into channel opening or closure. In electrically excitable cells such as neurons, the fast upstroke (membrane depolarizing phase) of the action potential (AP) is generally carried by an inward sodium or calcium current, whereas K v channels form the main repolarizing power that brings the membrane potential back to resting conditions and terminates the AP [1] . About 40 different K v subunits have been identified and since each displays unique channel kinetics they shape the AP in distinct ways [2] . The K v 3 subfamily contains four members; all four share the typical K v channel topology and are composed of four individual α-subunits, each containing six transmembrane helices (S1–S6) organized to form a central ion pore made by the S5 and S6 segments [3] . The channel’s main activation gate, which seals off the potassium pathway, is located at the bundle crossing region of the S6 segments [4] , [5] and is under control of the four VSDs comprised by the S1 through S4 helices. K v 3.1 and K v 3.2 are delayed rectifiers while K v 3.3 and K v 3.4 yield transient outward currents because of rapid N-type inactivation involving the N-terminus [6] , [7] , [8] . Despite their differences in inactivation behaviour they distinguish themselves from other K v channels by their positively shifted voltage dependence of channel opening and very fast deactivation kinetics [9] . These unique properties make K v 3 channels suited for their job in neurons that fire short duration APs at high frequencies [10] , [11] . The positively shifted voltage dependence of K v 3 channel opening sets a low threshold for AP initiation and, in combination with fast deactivation kinetics, minimizes the after-hyperpolarization such that the initiation and height of subsequent APs are not compromised. Thus, the behaviour of K v 3 channels is conducive to short AP intervals and sustainable high-frequency AP transmission. Although K v 3 channels are abundantly expressed in the central nervous system as a whole, they are enriched in subsets of fast-spiking interneurons, rapidly firing cerebellar Purkinje cells, and central auditory nuclei where neurons can follow high-frequency input [12] , [13] , [14] , [15] , [16] , [17] , [18] , [19] , [20] , [21] , [22] . Because of their positively shifted voltage dependence of channel opening, K v 3 channels are mainly closed during rest and the AP upstroke. Therefore, they will only activate during the AP’s repolarization phase [9] . However, during brief APs, with a half-life duration as short as 100 μs [23] , the membrane potential remains more positive than the threshold for K v 3 channel activation, that is, −10 mV, for only a very short time. This raises the possibility that the K v 3 current will be insufficient to properly repolarize the membrane. The very rapid deactivation of K v 3 channels further exacerbates this problem. Thus, the known properties of the K v 3 channels raise the question of whether enough channels can open during the brief depolarization phase of the AP to generate sufficient current to repolarize the membrane potential completely [24] . If not, early after-depolarizations might occur, and the shape of successive APs within a pulse train might change or the train of APs could terminate early. One way to minimize the risk of insufficient repolarization during high-frequency AP firing is to express high quantities of K v 3 channels to ensure that sufficient channels are active during the repolarization phase [9] . Here we report an additional solution: K v 3.1b channels have a built-in safety mechanism in their gating kinetics that favours channel opening during membrane repolarization. This novel safety mechanism allows channels that reach an intermediate transition to open instead of deactivating during repolarization. This produces a resurgent K + current (or hooked tail) that provides an extra impediment to the potential failure of rapidly firing neurons to repolarize. While resurgent currents are also found in voltage-gated sodium (Na v ) channels [25] and the human Ether-a-gogo-related (hERG) K v channel [26] , [27] , these have been shown to originate due to recovery from open-channel block, induced by the cytoplasmic tail of the β4 subunit [28] or extremely rapid recovery from channel inactivation [29] , [30] , respectively. The resurgent K + current reported here for K v 3.1b is driven through a process distinct from either of these, but can similarly be described as a resurgent current. In Shaker-type K v channels, the stabilization of the VSD in its active state, through a process termed relaxation, is a slow process that develops after channel opening [31] . In contrast, the VSD in K v 3.1b channels relaxes extremely quickly, even preceding channel opening. This rapid relaxation process results in a deceleration of the deactivation kinetics on very brief depolarizations; in turn, the slowing of the deactivation kinetics results in a resurgent K + current upon membrane repolarization. Introducing this feature in a simple Markov state model was sufficient to simulate the resurgent K + current, further suggesting that the underlying mechanism for the resurgent current in K v 3.1b channels is the relative speed of channel deactivation compared with activation. VSD relaxation in Kv3.1b precedes channel gate opening In K v channels, the membrane potential is detected by the VSD, which contains the positively charged S4 segment. Changes in membrane potential result in a VSD motion that displaces the electrical charges on the S4 segment (gating charges) within the membrane electric field and can therefore be detected as a transient gating current [32] . It has been demonstrated that S4-based VSDs with a four-transmembrane topology display relaxation, a process that stabilizes the VSDs in their active state [33] . In the case of Shaker-type K v channels, the VSD relaxes after the channel opens and manifests itself as a slowing down in VSD deactivation [31] , [34] . Because of the tight coupling with the channel gate, this VSD relaxation is reflected in slower closure times of the channel gate [34] . As the mechanism of VSD relaxation is probably a general behaviour in this class of VSDs, it is conceivable that a similar mechanism is present in K v 3.1b channels. If the VSD of K v 3.1b indeed relaxes and this process develops after the channel gate opens as in Shaker, prolonged depolarization times (or gradual accumulation during bursts of AP firing) should slow down channel closure which would impair the AP firing pattern [10] . To this end, gating currents were recorded from wild-type (WT) conducting K v 3.1b channels (detailed steady-state ionic current data of K v 3.1b is provided in Supplementary Fig. 1 ). Gating currents were detectable after depleting the oocytes of K + by repetitive activation of the channels followed by external TEA (tetra-ethyl-ammonium) application to block the remaining ionic current ( Fig. 1a,b ). To determine the voltage dependence of VSD activation, gating currents were elicited by pulsing from a constant hyperpolarized initial voltage to more positive voltages (activation protocol, Fig. 1a ). To obtain the voltage dependence of VSD deactivation, deactivating (Ig deac ) gating currents were generated by pulsing from a constant positive voltage to more negative voltages (deactivation protocol, Fig. 1b ). The typical charge (Q) versus voltage QV curve was obtained by integrating the off (Ig off ) gating currents of an activation protocol, yielding a QV curve with an average midpoint value±s.e.m. of 6.2±1.6 mV ( n =6) and a valence z of 3.9±0.2 mV ( Fig. 1c ). For comparison, the GV curve is also plotted in Fig. 1c . The time constant of the decaying phase of the gating current, Ig ac, ( τ Igac ) nicely matched the time constant of ionic current activation τ Iiac ( Fig. 1d ), as was reported for Shaker [34] . In Shaker, the ionic Ii deac kinetics ( τ Iideac ) were typically faster than the Ig deac kinetics ( τ Igdeac ); this behaviour was also observed in K v 3.1b in the voltage window of −50 to −140 mV ( Fig. 1d ). In the voltage range between 0 and −40 mV, however, τ Iideac was slower than τ Igdeac , likely because τ Igdeac slows down such that its amplitude becomes too small to be resolved from the electric noise (see Supplementary Fig. 2 for more details). 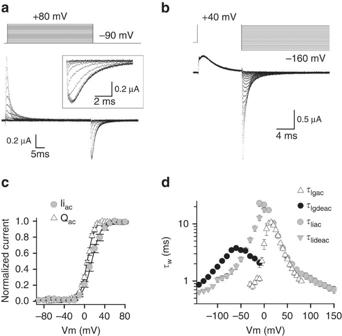Figure 1: Kv3.1b gating current recordings monitor the VSD movement. (a) Gating currents (Ig) of WT Kv3.1b after depletion of K+and subsequent application of external TEA to block the remaining ionic current. Ig recordings were obtained using the activation pulse protocol shown on top. The holding potential was −120 mV and cells were depolarized in 5-mV increments from −120 mV to +80 mV. Background leak and capacitive currents were subtracted using a –P/4 protocol. Inset shows a scaled-up view of the Igoffcurrents obtained by stepping to −90 mV. (b) Pulse protocol to analyse the deactivating Igdeaccurrents. (c) Voltage dependence of activating charge movement (QV curve, open triangles), which was obtained by integrating the Igoffcurrents from pulse protocols shown ina(data are shown as average±s.e.m.,n=6). For comparison, the ionic GV curve fromSupplementary Fig. 1is displayed (grey circles). (d) Voltage dependence of the average time constants±s.e.m. of Igac(τIgac, open triangles,n=6) and Igdeac(τIgdeac, black circles,n=6).τIgackinetics were obtained from fitting the Igaccurrent decays (from pulse protocols shown ina) with a single exponential function.τIgdeackinetics were obtained by approximating the Igdeaccurrent decays (from pulse protocols shown inb) with a double exponential function and represented values are the weighted time constants. As comparison the ionicτIiacandτIideackinetics (Supplementary Fig. 1) are displayed in grey circles and triangles, respectively. Figure 1: K v 3.1b gating current recordings monitor the VSD movement. ( a ) Gating currents (Ig) of WT K v 3.1b after depletion of K + and subsequent application of external TEA to block the remaining ionic current. Ig recordings were obtained using the activation pulse protocol shown on top. The holding potential was −120 mV and cells were depolarized in 5-mV increments from −120 mV to +80 mV. Background leak and capacitive currents were subtracted using a –P/4 protocol. Inset shows a scaled-up view of the Ig off currents obtained by stepping to −90 mV. ( b ) Pulse protocol to analyse the deactivating Ig deac currents. ( c ) Voltage dependence of activating charge movement (QV curve, open triangles), which was obtained by integrating the Ig off currents from pulse protocols shown in a (data are shown as average±s.e.m., n =6). For comparison, the ionic GV curve from Supplementary Fig. 1 is displayed (grey circles). ( d ) Voltage dependence of the average time constants±s.e.m. of Ig ac ( τ Igac , open triangles, n =6) and Ig deac ( τ Igdeac , black circles, n =6). τ Igac kinetics were obtained from fitting the Ig ac current decays (from pulse protocols shown in a ) with a single exponential function. τ Igdeac kinetics were obtained by approximating the Ig deac current decays (from pulse protocols shown in b ) with a double exponential function and represented values are the weighted time constants. As comparison the ionic τ Iiac and τ Iideac kinetics ( Supplementary Fig. 1 ) are displayed in grey circles and triangles, respectively. Full size image To test whether K v 3.1b channels display VSD relaxation, Ig deac kinetics ( τ Igdeac ) were determined upon different activating pulse durations at +40 mV, which varied from 0.3 ms (the shortest) to 10 s (the longest) in duration ( Fig. 2 ). Prolonging the duration of depolarization showed that K v 3.1b displayed a fast deceleration in its τ Igdeac kinetics, which developed within a time window of 0.3 to 2 ms ( Fig. 2a,b ). When the activating pulse duration was extended up to 10 ms, there was a second noticeable slowing in the τ Igdeac kinetics ( Fig. 2c,d ). However, as opposed to what had been seen in Shaker-type K v channels [34] , longer depolarization times (up to 10 s) did not result in an extra slowing down of the τ Igdeac kinetics. Thus, a VSD relaxation process as occurs in Shaker-type K v channels is not present in K v 3.1b, and prolonged depolarizations (longer than 10 ms) will not slow down the VSD deactivation kinetics and impair repetitive AP firing. 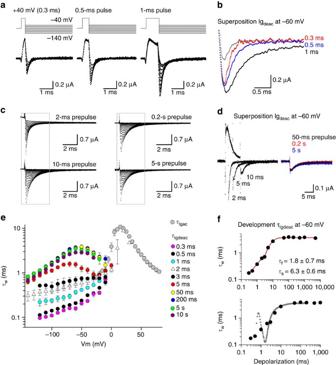Figure 2: Igdeackinetics of Kv3.1b as a function of activating pulse duration. (a) Igdeaccurrents upon very short depolarizations to +40 mV elicited using the pulse protocol shown on top. (b) Superposition of Igdeacrecordings fromaat −60-mV repolarization following a 0.3-ms (grey, with a scaled version shown in red), a 0.5-ms (blue) and a 1-ms (black) long activating pulse to +40 mV. Note the gradual deceleration in Igdeacwith increasing pulse duration. (c) Igdeaccurrents on different pulse durations at +40 mV (2 ms to 5 s in duration). The protocols were applied in a random order to exclude non-specific or depletion artifacts that might affect the kinetics over time, such as depletion of PIP2 levels57. (d) Left, superposition of Igdeacat −60 mV following 2-, 5- and 10-ms-long activating pulses. Right, superposition of Igdeacat −60 mV following 50-ms (black), 0.2-s (red) and 5-s (blue) long activating pulses. Prolonging the pulse from 2 to 10 ms slowed down Igdeacdecay further whereas longer pulses had no additional effect. (e) Voltage dependence of the weightedτIgdeactime constants as a function of activating pulse duration. Data is shown as mean±s.e.m. (n=5). Note the gradual slowing inτIgdeacwhen depolarization times became longer. (f) Top panel shows the mean±s.e.m. of the weightedτIgdeactime constant at −60 mV as a function of depolarization time (n=5). This plot shows that there are two slowing processes, and fitting this relation with a double exponential function indicated that the deceleration inτIgdeacdeveloped with a fast time constant (τf) of 1.8±0.7 ms and a slower component (τs) of 6.3±0.6 ms (n=5). The bottom panel displays a superposition of the same Igdeackinetics and a scaled ionic current activation (the first spike in ionic current trace is the remaining capacitive transient). Note that the second slowing process (τs) matched the time course of channel opening. Figure 2: Ig deac kinetics of K v 3.1b as a function of activating pulse duration. ( a ) Ig deac currents upon very short depolarizations to +40 mV elicited using the pulse protocol shown on top. ( b ) Superposition of Ig deac recordings from a at −60-mV repolarization following a 0.3-ms (grey, with a scaled version shown in red), a 0.5-ms (blue) and a 1-ms (black) long activating pulse to +40 mV. Note the gradual deceleration in Ig deac with increasing pulse duration. ( c ) Ig deac currents on different pulse durations at +40 mV (2 ms to 5 s in duration). The protocols were applied in a random order to exclude non-specific or depletion artifacts that might affect the kinetics over time, such as depletion of PIP2 levels [57] . ( d ) Left, superposition of Ig deac at −60 mV following 2-, 5- and 10-ms-long activating pulses. Right, superposition of Ig deac at −60 mV following 50-ms (black), 0.2-s (red) and 5-s (blue) long activating pulses. Prolonging the pulse from 2 to 10 ms slowed down Ig deac decay further whereas longer pulses had no additional effect. ( e ) Voltage dependence of the weighted τ Igdeac time constants as a function of activating pulse duration. Data is shown as mean±s.e.m. ( n =5). Note the gradual slowing in τ Igdeac when depolarization times became longer. ( f ) Top panel shows the mean±s.e.m. of the weighted τ Igdeac time constant at −60 mV as a function of depolarization time ( n =5). This plot shows that there are two slowing processes, and fitting this relation with a double exponential function indicated that the deceleration in τ Igdeac developed with a fast time constant (τf) of 1.8±0.7 ms and a slower component (τs) of 6.3±0.6 ms ( n =5). The bottom panel displays a superposition of the same Ig deac kinetics and a scaled ionic current activation (the first spike in ionic current trace is the remaining capacitive transient). Note that the second slowing process (τs) matched the time course of channel opening. Full size image To quantify the dependency of the deceleration in τ Igdeac on the duration of the activating pulse, the decays of the Ig deac currents were fitted with a double exponential function and the weighted τ Igdeac time constants were plotted as a function of repolarizing voltage ( Fig. 2e ). This analysis emphasized that Ig deac decay slowed down as a function of activating step duration. When we plotted the weighted τ Igdeac time constants at −60 mV as a function of depolarization time ( Fig. 2f ), there were two identifiable decelerations of the τ Igdeac kinetics when the activating pulse durations at +40 mV were increased from 0.3 ms up to ∼ 50 ms. Compared with the time constant of ionic current activation, which at +40 mV amounts to 3.8±0.2 ms ( n =9) ( Supplementary Fig. 1 ), the first slowing in τ Igdeac appeared to develop before the channel opened. Indeed, plotting a scaled ionic Ii ac current activation on top of the relation between τ Igdeac and activating pulse duration demonstrated that the second slowing in τ Igdeac matched channel opening whereas the first slowing preceded it ( Fig. 2f ). Although we cannot fully exclude that VSD relaxation in K v 3.1b channels is extremely slow with a time constant longer than 10 s or in the extreme case even absent, we propose that the fast-developing slowing of the τ Igdeac kinetics of K v 3.1b corresponds to VSD relaxation that precedes channel gate opening. VSD relaxation slows the deactivation of a pre-active state For Shaker-type K v channels it is well-documented that channel gate opening induces a deceleration in τ Igdeac (ref. 35 ). At the molecular level, this deceleration is caused by the establishment of intra-subunit interactions between residues of the S4–S5 linker and C-terminal S6 segment [36] , [37] . Because of the strong interaction between VSD movements and channel gate rearrangements [38] , this deceleration in τ Igdeac is accompanied by a similar slowing in the τ Iideac closure times of the channel gate of Shaker-type K v channels [34] . In K v 3.1b, channel gate opening most likely accounts for the second slowing in τ Igdeac , based on the overlap between channel gate opening and the onset of the second deceleration of τ Igdeac kinetics ( Fig. 2f ). Consequently, a similar slowing should be detected in the kinetics of channel gate closure as a function of activating step duration. Plotting the voltage-dependent Ii deac time constants ( τ Iideac ) on different activating pulse durations at +40 mV indicated that there was a small but identifiable slowing in the τ Iideac kinetics ( Fig. 3a,b ). When the weighted τ Iideac time constant at −60 mV was plotted as a function of activating pulse duration there was, in contrast to the VSD deactivation ( τ Igdeac ) behaviour, only a single noticeable slowing process in the τ Iideac kinetics ( Fig. 3c,d ). This deceleration in τ Iideac developed with a time constant of 6.6±1.7 ms ( n =5) and matched the time constant of the second slowing process in τ Igdeac kinetics ( Fig. 2f ). On the other hand, the fast-developing deceleration process in the τ Igdeac kinetics of K v 3.1b was not reflected in the speed of channel gate closure ( τ Iideac ), which is further evidence that this fast-developing deceleration of VSD deactivation occurs prior to the gate opening of the channel. 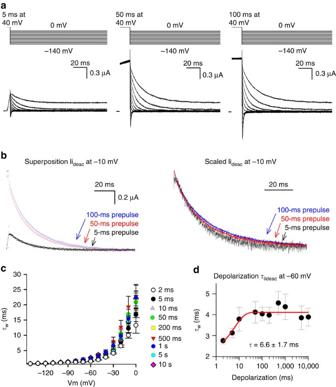Figure 3: Iideackinetics of Kv3.1b as a function of activating pulse duration. (a) Ionic current deactivation (Iideac) of Kv3.1b elicited using the pulse protocols shown on top. From left to right the activating pulse at +40 mV was increased from 5 to 50 ms, and to 100 ms. (b) Left panel shows a superposition of Iideacat −10 mV following a 5-ms (black), a 50-ms (red) and a 100-ms (blue) long activating pulse. Right panel displays a superposition of the same Iideaccurrents after rescaling them. Note the slowing in Iideacdecay time (τIideac) when the duration of the activating pulse was increased. (c) Voltage dependence of the weightedτIideacas a function of activating pulse duration at +40 mV, shown as mean±s.e.m. (n=5). When the duration time was increased from 2 ms (white) up to 50 ms (green) there was a gradual deceleration inτIideac. Note that depolarizations longer than 50 ms in duration did not cause any further significant changes inτIideac. (d) WeightedτIideacat −60 mV as a function of depolarization time. This plot shows, in contrast to Igdeackinetics, that the Iideackinetics displayed only a single slowing process, which developed with a time constant of 6.6±1.7 ms (n=5, data represented as mean±s.e.m.). Figure 3: Ii deac kinetics of K v 3.1b as a function of activating pulse duration. ( a ) Ionic current deactivation (Ii deac ) of K v 3.1b elicited using the pulse protocols shown on top. From left to right the activating pulse at +40 mV was increased from 5 to 50 ms, and to 100 ms. ( b ) Left panel shows a superposition of Ii deac at −10 mV following a 5-ms (black), a 50-ms (red) and a 100-ms (blue) long activating pulse. Right panel displays a superposition of the same Ii deac currents after rescaling them. Note the slowing in Ii deac decay time ( τ Iideac ) when the duration of the activating pulse was increased. ( c ) Voltage dependence of the weighted τ Iideac as a function of activating pulse duration at +40 mV, shown as mean±s.e.m. ( n =5). When the duration time was increased from 2 ms (white) up to 50 ms (green) there was a gradual deceleration in τ Iideac . Note that depolarizations longer than 50 ms in duration did not cause any further significant changes in τ Iideac . ( d ) Weighted τ Iideac at −60 mV as a function of depolarization time. This plot shows, in contrast to Ig deac kinetics, that the Ii deac kinetics displayed only a single slowing process, which developed with a time constant of 6.6±1.7 ms ( n =5, data represented as mean±s.e.m.). Full size image Comparing the Ii deac and Ig deac behaviour as a function of activating pulse duration, it became evident that the VSD of K v 3.1b channels can relax (or reach an equivalent stabilized active state) from a non-conducting pre-active channel configuration. To test this further, we monitored the behaviour of the τ Igdeac kinetics in the presence of 4-aminopyridine (4-AP). K v 3 channels are highly sensitive to 4-AP which binds in the channel pore [39] and inhibits the channel by stabilizing the non-conducting pre-active state [40] , [41] . Consequently, 4-AP is the appropriate pharmacological tool to investigate whether reaching the pre-active state is sufficient for K v 3.1b channels to have VSD relaxation. Studying the Ig deac behaviour of K v 3.1b channels in presence of 1 mM 4-AP, a concentration that induces full channel inhibition, showed that the decay time slowed down when the activating pulse at +40 mV was prolonged from 0.3 to 10 ms in duration ( Fig. 4a,b ). Plotting the average weighted τ Igdeac time constants upon different activating pulse durations confirmed a clear depolarization-dependent slowing in the Ig deac kinetics ( Fig. 4c ). This deceleration was better illustrated by plotting the weighted τ Igdeac time constant at −60 mV as a function of depolarization time ( Fig. 4d ). The slowing developed quite quickly and displayed a time constant of 2.7±0.4 ms ( n =5), which matched the first fast-developing deceleration in Ig deac kinetics observed in the absence of 4-AP. However, the second deceleration process in the Ig deac kinetics was prevented by 4-AP, which further suggests that this slowing in VSD deactivation developed via channel gate opening. 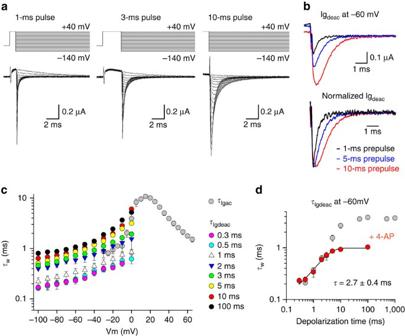Figure 4: Kv3.1b relaxes from a pre-active state in the presence of 4-AP. (a) Igdeaccurrents of Kv3.1b in the presence of 1 mM 4-aminopyridine (4-AP) with different activating pulse durations at +40 mV. (b) Top panel, superposition of Igdeacat −60 mV on a 1-ms (black), 5-ms (blue) and 10-ms (red) long depolarization to +40 mV. Bottom panel, superposition of the same Igdeaccurrents after normalization. Note the gradual deceleration in Igdeacdecay as the activating pulses are prolonged. (c) Igdeackinetics (τIgdeac) as a function of depolarization time in the presence of 1 mM 4-AP, displayed as mean±s.e.m. (n=5). Even in the presence of 1 mM 4-AP there was a noticeable deceleration inτIgdeacthat developed relatively quickly. For example, compareτIideacon a 0.3-ms (pink) and a 3-ms (green) activating pulse at+40 mV. (d) WeightedτIgdeacat −60 mV as a function of the activating pulse duration in both the absence (grey) and presence of 1 mM 4-AP (red), shown as mean±s.e.m. (n=5).τIgdeacwas slowed down in presence of 4-AP, a deceleration that developed over a similar time window as the fast slowing process (τf) in control conditions. Figure 4: K v 3.1b relaxes from a pre-active state in the presence of 4-AP. ( a ) Ig deac currents of K v 3.1b in the presence of 1 mM 4-aminopyridine (4-AP) with different activating pulse durations at +40 mV. ( b ) Top panel, superposition of Ig deac at −60 mV on a 1-ms (black), 5-ms (blue) and 10-ms (red) long depolarization to +40 mV. Bottom panel, superposition of the same Ig deac currents after normalization. Note the gradual deceleration in Ig deac decay as the activating pulses are prolonged. ( c ) Ig deac kinetics ( τ Igdeac ) as a function of depolarization time in the presence of 1 mM 4-AP, displayed as mean±s.e.m. ( n =5). Even in the presence of 1 mM 4-AP there was a noticeable deceleration in τ Igdeac that developed relatively quickly. For example, compare τ Iideac on a 0.3-ms (pink) and a 3-ms (green) activating pulse at+40 mV. ( d ) Weighted τ Igdeac at −60 mV as a function of the activating pulse duration in both the absence (grey) and presence of 1 mM 4-AP (red), shown as mean±s.e.m. ( n =5). τ Igdeac was slowed down in presence of 4-AP, a deceleration that developed over a similar time window as the fast slowing process (τf) in control conditions. Full size image Collectively, this data is consistent with the view that the VSD of K v 3.1b channels relaxes before the channel gate opens. This relaxation-induced stabilization consequently slows down the deactivation kinetics from a non-conducting pre-active state, which most likely also affects channel gate opening and closing on brief depolarizing pulses. Thus, during brief depolarizing pulses, the VSDs of K v 3.1b channels enter the relaxed state; this slows the return of the VSD to the resting state during a subsequent hyperpolarizing pulse. This stabilization of a non-conducting pre-active state most likely also affects channel gate opening and closing upon brief depolarizing pulses. K v 3.1b channels display a timely resurgent K + current If this fast-developing VSD relaxation process is relevant for Kv3.1b’s function in vivo , its impact would be manifested on non-steady-state activations whereby a substantial amount of the channels populate the non-conducting pre-active state. To investigate this, we studied K v 3.1b deactivation kinetics upon brief activating, that is, depolarizing, pulses. Remarkably, upon short activating pulses, which are insufficient to have full channel opening (that is, being in non-steady-state conditions), K v 3.1b channels displayed a marked resurgent K + (hooked tail) current during the subsequent repolarization to potentials that close the channel ( Fig. 5a ). These brief activating pulses reflect more closely the physiological situation as K v 3.1b channels most likely do not reach steady-state activation during the brief depolarization phase of the neuronal AP [9] , [24] , [42] . With a longer activation pulse, which induces steady-state channel activation, a resurgent K + current was not observed ( Fig. 5b ). In contrast, Shaker, which undergoes VSD relaxation after the channel gate opens, never displayed a hooked tail current on short pulses ( Fig. 5c ). 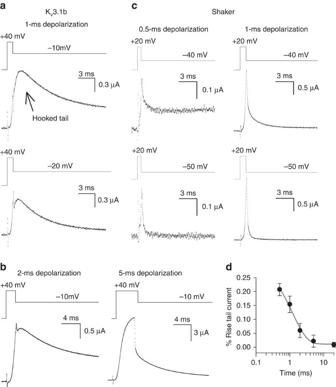Figure 5: Kv3.1b displays a hooked ionic tail current on short activating pulses. (a) Kv3.1b deactivating ionic currents on a 1-ms activating pulse to +40 mV. A resurgent K+(hooked tail) current was observed on the subsequent repolarization to potentials below the threshold for channel opening, which localizes around −10 mV (Supplementary Fig. 1c). (b) Kv3.1b deactivating ionic currents on a 2-ms (left panels) or a 5-ms (right panels) activating pulse to +40 mV. When the activating pulse was prolonged (for example, 5 ms), the resurgent K+current disappeared gradually. See alsoSupplementary Fig. 3. (c) Deactivating ionic currents (Iideac) of the Shaker channel using similar pulse protocols. Since theτIiackinetics of Shaker are slightly faster than those of Kv3.1b, even shorter activating pulses were applied. However, in contrast to Kv3.1b, the Shaker channel never displayed a hooked tail current even on activating pulses as short as 0.5 ms (left panels) or 1 ms (recordings on the right). (d) Normalized amplitude of the resurgent K+current in Kv3.1b on a repolarization to −10 mV as a function of activating pulse duration. On very short activating pulses (for example, 0.5 ms), the amplitude of the hooked tail amounted to∼23% of the total tail current amplitude. When the duration of the activating pulse was prolonged, the amplitude of the resurgent K+current decreased exponentially with a time constant of 1.7±0.8 ms (grey line,n=5, data represented as mean±s.e.m.). Figure 5: K v 3.1b displays a hooked ionic tail current on short activating pulses. ( a ) K v 3.1b deactivating ionic currents on a 1-ms activating pulse to +40 mV. A resurgent K + (hooked tail) current was observed on the subsequent repolarization to potentials below the threshold for channel opening, which localizes around −10 mV ( Supplementary Fig. 1c ). ( b ) K v 3.1b deactivating ionic currents on a 2-ms (left panels) or a 5-ms (right panels) activating pulse to +40 mV. When the activating pulse was prolonged (for example, 5 ms), the resurgent K + current disappeared gradually. See also Supplementary Fig. 3 . ( c ) Deactivating ionic currents (Ii deac ) of the Shaker channel using similar pulse protocols. Since the τ Iiac kinetics of Shaker are slightly faster than those of K v 3.1b, even shorter activating pulses were applied. However, in contrast to K v 3.1b, the Shaker channel never displayed a hooked tail current even on activating pulses as short as 0.5 ms (left panels) or 1 ms (recordings on the right). ( d ) Normalized amplitude of the resurgent K + current in K v 3.1b on a repolarization to −10 mV as a function of activating pulse duration. On very short activating pulses (for example, 0.5 ms), the amplitude of the hooked tail amounted to ∼ 23% of the total tail current amplitude. When the duration of the activating pulse was prolonged, the amplitude of the resurgent K + current decreased exponentially with a time constant of 1.7±0.8 ms (grey line, n =5, data represented as mean±s.e.m.). Full size image When a resurgent K + current was present, the derivative at the initial tail current value, immediately following the application of the repolarizing potential, was positive. To determine the contribution of this resurgent K + current to K v 3.1b’s total tail current amplitude, we determined the maximal tail current amplitude and normalized it to the initial tail current value. In this way, we obtained the percentage rise in tail current amplitude (that is, quantified the amplitude of the resurgent K + current). At a repolarizing potential of −10 mV following a 1-ms activation pulse ( Fig. 5a ), the contribution of the resurgent current was about 25% of the total current amplitude ( Fig. 5d ). When the activation pulse exceeded 2 ms ( Fig. 5b ), the initial tail current value was the maximum tail current amplitude and the contribution of the resurgent K + current was consequently about 0% ( Fig. 5d ). Plotting the percentage rise of the tail current amplitude as a function of activating pulse duration clearly showed that the resurgent tail current decreased in amplitude when the activation pulses were prolonged ( Fig. 5d ). Thus, the resurgent K + current was gradually lost, and absent when activation pulses were sufficiently long to have full channel opening. This analysis emphasized that the occurrence of a resurgent K + current in K v 3.1b was a temporal feature elicited on non-steady-state activation only. Since a resurgent K + (hooked tail) current during channel deactivation yields a transient increase in repolarizing power, this feature might secure membrane repolarization during the falling phase of the AP that normally works as a negative feedback on channel closure. The well-described resurgent K + current of the hERG channel originates from the channel’s particular inactivation mechanism [27] , [30] . During channel opening, the hERG channel quickly undergoes inactivation, a process whereby the K + pathway becomes non-conducting although the channel gate remains open, and only a fraction of the hERG channels conduct K + ions. Since upon repolarization the time course of recovery from their inactive state is faster than channel gate closure, inactive channels are recruited to their open conducting state before closing. Therefore, hERG channels always display a resurgent K + current independent of the activating depolarization time [29] , [30] . If the resurgent K + current in K v 3.1b originated from a similar underlying inactivation mechanism, the resurgent current would remain when depolarization times were prolonged. However, this was not the case and the hooked tail disappeared when the depolarization time of the activating pulse was increased ( Fig. 5b,d ; Supplementary Fig. 3 ). Therefore, K v 3.1b channels distinguish themselves from the hERG channel; a different mechanism generates the resurgent K + current in K v 3.1b. K v 3.1b’s unique S3–S4 linker mediates its resurgent K + current The resurgent K + current of K v 3.1b channels on short activating pulses seems driven by an accelerated transition into the VSD relaxed state, an acceleration that does not exist in the Shaker channel. In a search to identify possible molecular mediators of this difference, we looked at molecular determinants that control VSD relaxation. The entrance into the relaxed state could be accelerated in Shaker by shortening the VSD’s S3–S4 linker [43] . The S3–S4 linker sequence is highly conserved within the K v 3 family, and it is very different from those in other K v channels, including the Shaker K v channels ( Fig. 6a ). In Shaker, the S3–S4 linker length is 31 amino acids, based on prior investigations of the periodicity of the linker [44] . The homologous region in K v 3.1b channels is only 14 amino acids long ( Fig. 6a ). Furthermore, numerous prior reports had suggested that the S3–S4 linker modulates the kinetic and energetic properties of other K v channels, as well as voltage-dependent sodium and calcium channels [45] , [46] , [47] , [48] , [49] . 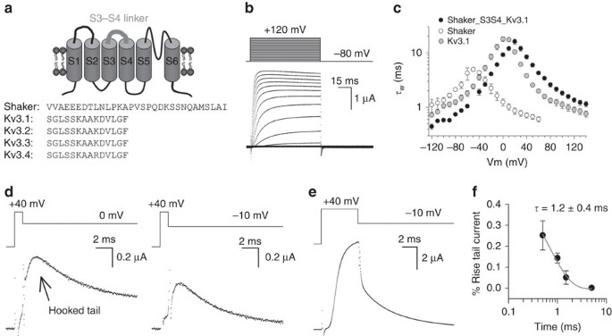Figure 6: A chimeric Shaker channel with Kv3.1b’s S3–S4 linker generates a resurgent K+current. (a) On top, a cartoon of the topology of a Kvα-subunit composed of six transmembrane segments (S1–S6) with the VSD’s S3–S4 linker highlighted in grey. Below a sequence alignment of the S3–S4 linker of Shaker and the different Kv3 family members. (b) Representative ionic Iiaccurrent recordings of the Shaker_S3S4_Kv3.1 chimera elicited with the pulse protocol shown on top. See alsoSupplementary Fig. 4. (c) Weighted time constants±s.e.m. of channel gate opening (τIiac,n=9) and closing (τIideac) for the Shaker_S3S4_Kv3.1 chimera (black circles,n=4). The time constants for Kv3.1b (grey) and Shaker (open) are taken fromFig. 1dand redisplayed as comparison. (d) Iideaccurrents of the Shaker_S3S4_Kv3.1 chimera elicited at 0 mV (left recording) and −10 mV (right recording) on a 1-ms activating pulse to +40 mV, respectively. On such brief activating pulses, the Shaker_S3S4_Kv3.1 chimera displayed a resurgent K+(hooked tail) current. (e) Iideacat −10 mV elicited on a 5-ms activating pulse to +40 mV. Note the absence of a resurgent K+current. (f) Normalized amplitude of the resurgent K+current on a repolarization to −10 mV as a function of activating pulse duration. The amplitude of the resurgent K+current was maximally about 25% of the total tail current amplitude, and decreased in amplitude when the activating pulse was prolonged (the loss of a resurgent K+current developed with a time constant of 1.2±0.4 ms,n=5, data shown as mean±s.e.m.). Figure 6: A chimeric Shaker channel with K v 3.1b’s S3–S4 linker generates a resurgent K + current. ( a ) On top, a cartoon of the topology of a K v α-subunit composed of six transmembrane segments (S1–S6) with the VSD’s S3–S4 linker highlighted in grey. Below a sequence alignment of the S3–S4 linker of Shaker and the different K v 3 family members. ( b ) Representative ionic Ii ac current recordings of the Shaker_S3S4_K v 3.1 chimera elicited with the pulse protocol shown on top. See also Supplementary Fig. 4 . ( c ) Weighted time constants±s.e.m. of channel gate opening ( τ Iiac , n =9) and closing ( τ Iideac ) for the Shaker_S3S4_K v 3.1 chimera (black circles, n =4). The time constants for K v 3.1b (grey) and Shaker (open) are taken from Fig. 1d and redisplayed as comparison. ( d ) Ii deac currents of the Shaker_S3S4_K v 3.1 chimera elicited at 0 mV (left recording) and −10 mV (right recording) on a 1-ms activating pulse to +40 mV, respectively. On such brief activating pulses, the Shaker_S3S4_K v 3.1 chimera displayed a resurgent K + (hooked tail) current. ( e ) Ii deac at −10 mV elicited on a 5-ms activating pulse to +40 mV. Note the absence of a resurgent K + current. ( f ) Normalized amplitude of the resurgent K + current on a repolarization to −10 mV as a function of activating pulse duration. The amplitude of the resurgent K + current was maximally about 25% of the total tail current amplitude, and decreased in amplitude when the activating pulse was prolonged (the loss of a resurgent K + current developed with a time constant of 1.2±0.4 ms, n =5, data shown as mean±s.e.m.). Full size image As the identities of the amino acids in the S3–S4 helix have been shown to alter K v channel activity [50] and shortening the S3–S4 linker accelerated the relaxation process [43] , we tested whether K v 3.1b’s unique S3–S4 linker sequence was a key determinant to produce the resurgent K + current. To this end, we substituted in both K v 3.1b and Shaker the S3–S4 linker with its reciprocal Shaker and K v 3.1b sequence, generating the channel chimeras K v 3.1_S3S4_Shaker and Shaker_S3S4_K v 3.1. Unfortunately, the K v 3.1_S3S4_Shaker chimera did not produce ionic currents in the voltage range of −130 to +180 mV ( Supplementary Fig. 4a ). On the other hand, expression of the reciprocal construct Shaker_S3S4_K v 3.1 chimera (that is, a Shaker channel with the S3–S4 linker substituted by the K v 3.1b sequence) produced robust ionic currents ( Fig. 6b ) that displayed a high threshold of channel activation, similar to WT K v 3.1b channels ( Supplementary Fig. 4b ). In addition, the steep voltage dependence in K v 3.1b’s ionic current kinetics ( Fig. 1 ; Supplementary Fig. 1 ), but absent in Shaker, was also seen in the Shaker_S3S4_K v 3.1 channel ( Fig. 6c ). Most interestingly, when subjected to the same protocol of brief activating depolarizations, the Shaker_S3S4_K v 3.1 chimera generated a resurgent K + current on the subsequent repolarizing pulse as WT K v 3.1b did ( Fig. 6d ). Similarly, the resurgent K + current was only observed upon non-steady-state channel activation and prolonging the duration of the activating pulse resulted in a gradual loss in resurgent K + current amplitude ( Fig. 6e,f ). To investigate the VSD behaviour of the Shaker_S3S4_K v 3.1, we inserted the W434F mutation [51] , which yields a non-conducting Shaker channel that facilitates the recording of gating currents without affecting the VSD relaxation process [31] . The Shaker_S3S4_K v 3.1 W434F chimera yielded robust gating currents using activation and deactivation protocols ( Supplementary Fig. 5 ). In the Shaker_S3S4_K v 3.1 W434F chimera, prolonging the duration of the activating pulse to +40 mV resulted, as expected, in a slowing in deactivation gating currents ( Supplementary Fig. 6 ). Most interestingly, this slowing in VSD deactivation partially preceded channel gate opening, suggesting that the VSD displayed an accelerated relaxation process as is the case in K v 3.1b. However, in addition to the main gating charge movement that opens the channel at depolarized potentials, as occurs in K v 3.1b channels, the chimera exhibited a fast activating gating current component at very negative potentials ( Supplementary Fig. 5 ; Supplementary Discussion ). The presence of this early gating charge component obscured the exact origin of the slowing processes and we cannot draw a firm conclusion regarding the development of VSD relaxation in this chimera. Nevertheless, the S3–S4 linker of K v 3.1b appeared to be a sufficient molecular mediator of the resurgent K + current. Our steady-state ionic current data agreed with previous reports of K v 3.1b being a high-voltage, fast activating and deactivating delayed rectifier K v channel ( Supplementary Fig. 1 ). In addition, based on the ionic and gating current kinetics, K v 3.1b displays a strong voltage dependence in its τ Ii and τ Ig time constants ( Fig. 1d , note the more narrow bell-shaped voltage dependence of the τ Ig and τ Ii kinetics compared with Shaker), which ensures that channel closure is markedly accelerated with progressively stronger membrane repolarization. These features make K v 3.1b (and other K v 3 channels) well-suited for repolarizing cells that are highly excitable [9] , [11] . As originally noted, the APs of sustainable high-frequency AP transmission are <1 ms in duration; this raised the question of whether K v 3.1b could be sufficiently activated to secure complete membrane repolarization [9] , [24] , [42] . We show that K v 3.1b channels display a resurgent K + tail current on non-steady-state activation that may bypass this problem. It is clear that a particular inactivation mechanism or recovery from open-channel block, as is the case for the hERG and Na v channel, did not generate the resurgent K + current in K v 3.1b channels. A feature by which K v 3.1b and Shaker_S3S4_K v 3.1 channels distinguish themselves from the Shaker-type K v channels, which do not display a resurgent K + current, is their rapidly developing VSD relaxation process that precedes channel opening. We sought to further demonstrate the role of rapid VSD relaxation in inducing the resurgent ionic current through computational state analysis. In Shaker-type K v channels, VSD relaxation is a slowly developing process which normally occurs after channel opening, and the channels follow the activation sequence from pre-active non-conducting to active conducting and then to relaxed conducting ( Fig. 7a ), as proposed previously [34] . In contrast, K v 3.1b channels follow the activation sequence from pre-active to non-conducting, pre-active-relaxed and then to the conducting active-relaxed state ( Fig. 7a ). 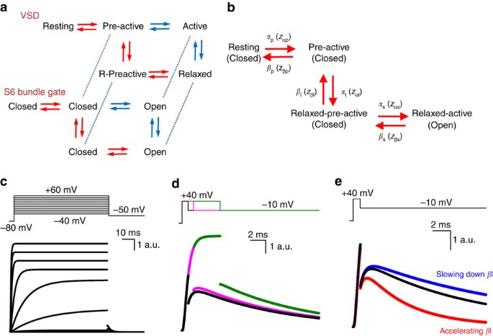Figure 7: A Markov model recapitulates a resurgent K+current based on a deceleration of VSD return. (a) A simplified state model of the VSD and pore, modified from ref.34. For clarity, we have excluded the open stabilized state that is linked to channel gate opening. The proposed pathway followed by the Shaker channel is highlighted in blue, while that followed by the Kv3.1b channel is in red. (b) Four-state Markov model of the voltage-sensing domain of Kv3.1b with three non-conducting and one conducting state (channel gate status is represented below between parentheses). The rate constants and valences of the different state transitions are represented inSupplementary Table 1. (c) The four-state Markov model depicted inbcould recapitulate Kv3.1b ionic current activations well using parameters based on experimental data (see Methods andSupplementary Table 1). (d) Under simulation of activation pulse protocols that produce resurgent K+currents experimentally, resurgent K+ionic currents were also generated by this four-state model (black trace, 0.8 ms). As in experimental results, extending the duration of the depolarizing pulse dramatically reduced the resurgent K+current (pink trace, 1.5 ms; green trace, 5 ms). (e) A threefold acceleration of the rate of return from the relaxed state (βl) with respect to the reference trace (black) reduced this resurgent K+current (red trace), while slowing the rate of return enhanced it (blue trace), suggesting that this is a critical parameter by which the resurgent K+current in Kv3.1b is generated in this model. For exact rate constants, please seeSupplementary Table 1. Figure 7: A Markov model recapitulates a resurgent K + current based on a deceleration of VSD return. ( a ) A simplified state model of the VSD and pore, modified from ref. 34 . For clarity, we have excluded the open stabilized state that is linked to channel gate opening. The proposed pathway followed by the Shaker channel is highlighted in blue, while that followed by the K v 3.1b channel is in red. ( b ) Four-state Markov model of the voltage-sensing domain of K v 3.1b with three non-conducting and one conducting state (channel gate status is represented below between parentheses). The rate constants and valences of the different state transitions are represented in Supplementary Table 1 . ( c ) The four-state Markov model depicted in b could recapitulate K v 3.1b ionic current activations well using parameters based on experimental data (see Methods and Supplementary Table 1 ). ( d ) Under simulation of activation pulse protocols that produce resurgent K + currents experimentally, resurgent K + ionic currents were also generated by this four-state model (black trace, 0.8 ms). As in experimental results, extending the duration of the depolarizing pulse dramatically reduced the resurgent K + current (pink trace, 1.5 ms; green trace, 5 ms). ( e ) A threefold acceleration of the rate of return from the relaxed state (βl) with respect to the reference trace (black) reduced this resurgent K + current (red trace), while slowing the rate of return enhanced it (blue trace), suggesting that this is a critical parameter by which the resurgent K + current in K v 3.1b is generated in this model. For exact rate constants, please see Supplementary Table 1 . Full size image To evaluate if the deceleration of VSD return caused by relaxation produces a resurgent K + current, we built a simple four-state sequential Markov model to simulate K v 3.1b currents ( Fig. 7b ). This model allowed us to eliminate the effect of VSD relaxation computationally and evaluate the impact of this process on the overall simulated current behaviour. The state pathway is based on the pathway for K v 3.1b proposed in Fig. 7a , and valences and rate constants of this model were determined from the experimental data ( Supplementary Table 1 ). This model reproduced classic channel activation very well ( Fig. 7c ). Furthermore, our model predicted the presence of a resurgent K + current when activating pulses were short; the simulations matched our experimentally obtained ionic current quite well, with the resurgent K + current amplitude equal to roughly 15% of the total current following a depolarizing pulse duration of 0.8 ms ( Fig. 7a ). In addition, upon prolonged depolarization times the hooked tail disappeared in our simulations as was the case experimentally ( Fig. 7d ). These simulations confirm our experimental observation and show that a resurgent K + current was only present in non-steady-state conditions, when not all channels have reached their fully open state. Having generated a simple Markov model that could simulate our experimental data allowed us to eliminate VSD relaxation and evaluate its contribution in generating the resurgent K + current. Based on our detailed gating current analysis in K v 3.1b channels, VSD relaxation results in approximately threefold slowing of the τ Igdeac kinetics ( Fig. 2f ). In our model, this slowing is reflected in the deactivation rates of the non-conducting pre-active-relaxed state. Therefore, in the model, the effect of VSD relaxation was eliminated by accelerating this deactivation rate constant by threefold. This interference was sufficient to greatly reduce the generation of a resurgent K + current ( Fig. 7e ). Furthermore, enhancing the impact of VSD relaxation by slowing the relaxation rate by 1.5-fold made the resurgent K + current more pronounced ( Fig. 7e ). This computational analysis showed that with short activating pulses a deceleration of the deactivation rate from a non-conducting pre-active state generates the resurgent K + current. That is, because of the slowed deactivation rate the transition from non-conducting, pre-active to open is more rapid than the transition to the deactivated state. As the resurgent K + current originates from the relative speed of channel activation compared with deactivation, the resurgent K + current is only observed with repolarizations between 0 and −40 mV as the accelerated deactivation rates at stronger repolarizations favour channel closure. In our model, the channels do not need to pass through a conducting state to undergo deactivation. Instead, a proportion of the K v 3.1b channel population opens for the first time from a pre-activated state during repolarization, as a consequence of their rapid activation and their slowed deactivation. Thus, the mechanism of the resurgent K + current we observe is distinct from the previously observed mechanisms of resurgent Na + current and hERG resurgent K + current. In agreement with our proposed mechanism for the presence of a resurgent K + current in K v 3.1b channels, AP-waveform clamp experiments on K v 3.1b-expressing HEK239 cells highlighted that the K v 3.1b current achieved its maximum amplitude during the repolarization phase of the AP [9] , [11] . Thus, the K v 3.1b channel produces a resurgent K + current at the membrane potentials where repolarization would be most likely to fail without this extra repolarizing power, that is, between 0 and −40 mV, but not at more hyperpolarized potentials where the K v 3.1b channel closes rapidly to minimize the after-hyperpolarization. It has become evident that the relaxation process is a general behaviour of S4-based VSDs that slows down the return of the VSD to the closed state, reflected by a slowing in τ Igdeac kinetics. However, the impact of this process on the channel’s kinetics and the time period of development may differ substantially between K v channel subtypes and other membrane proteins with a similar VSD topology. In the K v 3.1b VSD, relaxation develops rapidly. This phenomenon alters the relationship between the deactivation and activation kinetics and promotes the presence of a resurgent K + current ( Figs 2 , 4 , 7 ). Consequently, on short depolarizations, which are insufficient to have full K v 3.1b channel opening, a substantial amount of channels populate the pre-active-relaxed state that primes the channels to open by slowing VSD deactivation. Therefore, part of the channels that are in their pre-active-relaxed state will still transition to the open configuration during the subsequent membrane repolarization before closing. Other molecular determinants besides VSD relaxation may partially contribute to K v 3.1b’s unique relationship between deactivation and activation kinetics that generates the resurgent K + tail current. In this regard, it remains to be seen how auxiliary subunits that interact with K v 3 channels, such as KCNE subunits [52] , [53] , influence K v 3 channels’ resurgent K + currents in native neurons. However, our described mechanism for a resurgent K + current in K v 3.1b channels is novel and clearly different from the well-characterized, inactivation-dependent mechanism in the hERG channel. In conclusion, we report that the unique gating kinetics of K v 3.1b, which are attributed to the unique S3–S4 linker sequence of its VSD, result in a resurgent K + current upon membrane repolarization when channels move from non-conducting pre-active states (that is, upon short activating pulses). As this S3–S4 linker is highly conserved between different members of the K v 3 family, the findings reported here on K v 3.1b likely extend to the other K v 3-type channels. The resurgent K + current generated by K v 3.1b bypasses the problem of insufficient repolarizing power during the falling phase of the AP, a phase that normally works as a negative feedback mechanism on K v channel closure, and makes K v 3.1b channels ideally suited for high-frequency AP firing in certain regions of the central nervous system [9] , [11] , [23] . Expression in Xenopus oocytes In this study, we used the human K v 3.1b splice variant [54] and the fast-inactivation-removed Shaker-H4-IR (Δ6–46) clone [55] . Channel complementary DNAs (cDNAs) were cloned into a pBSTA vector modified for enhanced expression in Xenopus oocytes [56] . cDNAs were linearized using a Not1 restriction enzyme (New England Biolabs Inc., Ipswich, MA) that cut at a unique restriction site located after the poly-A sequence. Linearized cDNAs were transcribed into cRNAs using a T7 RNA Ambion expression kit (Invitrogen, Carlsbad, CA). Five to 50 ng of cRNA were injected into mature (stages 5 and 6) Xenopus oocytes 4–24 h after surgical extraction from adult frogs in accordance with both protocol 71475 of the University of Chicago Institutional Animal Care and Use Committee, and approval 2011-35 from the ethical commission for animal use of the University of Antwerp. Injected oocytes were maintained before recordings in a standard oocyte solution containing 96 mM NaCl, 2 mM KCl, 1.8 mM CaCl 2 , 1 mM MgCl 2 and 10 mM HEPES at pH 7.5 supplemented with 50 μg ml −1 gentamicin for 2 to 6 days at 16 °C. Molecular biology The S3–S4 linker sequence of K v 3.1b was inserted into Shaker and vice versa , generating the Shaker_S3S4_K v 3.1 and K v 3.1_S3S4_Shaker, with a site-directed mutagenesis PCR reaction using ‘megaprimers’. These megaprimers were generated during a prior PCR reaction using two specifically designed primers: the forward primer had a 3′ end that complemented the N-terminal region of the S3–S4 linker of the donor channel, while its 5′ end complemented the C-terminal region of the S3 segment of the acceptor channel, and the reverse primer had a 3′ end that complemented the C-terminal region of the S3–S4 linker of the donor channel and a 5′ end that complemented the N-terminal region of the S4 segment of the acceptor channel. The PCR-generated megaprimers, consisting of the S3–S4 linker of the donor channel flanked by nucleotides complementary to the S3 and S4 segment of the acceptor channel, were purified from gel with the NucleoSpin Gel and PCR Clean-up Kit, (Macherey-Nagel, Bethlehem, PA) following agarose gel electrophoresis and used for the subsequent mutagenesis PCR. PCR fragments were amplified in Escherichia coli and afterwards isolated using the NucleoSpin Plasmid Kit (Macherey-Nagel). The final constructs were double-strand sequenced to verify their correctness and the absence of unwanted mutations. Electrophysiology and solutions Ionic and gating current recordings were obtained at room temperature with the Dagan CA-1B high performance oocyte clamp amplifier (Dagan Corporation, Minneapolis, MN) in the cut-open voltage-clamp set-up. Current recordings were digitized with an in-house-built acquisition system based on the a4d4 module in the SB6711 digital signal processing unit (Innovative Integration, Simi Valley, CA) at a sampling frequency ranging from 10 to 100 kHz after 5–20 kHz low pass filtering. Pulse protocols and data acquisition were controlled using in-house-developed software. Recording pipettes with a resistance of 0.8–1.5 MΩ were pulled from 1.5-mm borosilicate glass capillaries (World Precision Instruments inc., Sarasota, FL) using a P87 micropipette puller (Sutter Instruments, Novato, CA). For gating current recordings, capacitive transient currents were subtracted online using the P/−4 method for activation protocols (−120-mV holding potential) and P/+4 for deactivation protocols (+20-mV holding potential) when possible. For ionic current recordings, the external solution contained 11.5 mM K-MES (methylsulfonate), 103.5 mM NMG (N-methyl-D-glucamine)-MES, 2 mM Ca-MES and 10 mM HEPES, and the internal solution contained 115 mM K-MES, 2 mM EGTA and 10 mM HEPES both adjusted to pH 7.5 using MES. Gating currents of the K v 3.1b channel were recorded after depleting the oocytes of K + by repetitive activation of the channels in continued perfusion of external NMG solution that lacks K + . Any remaining ionic current contamination was eliminated by external TEA block and the external recording solution contained 115 mM TEA-MES, 2 mM Ca-MES and 10 mM HEPES adjusted to pH 7.5 using MES. Gating current recordings of the Shaker_S3S4_K v 3.1 chimera were done in the W434F mutant [51] , which abolishes K + conduction, and using an external NMG-MES solution that contained 115 mM NMG-MES, 2 mM Ca-MES and 10 mM HEPES adjusted to pH 7.5 using MES. For both K v 3.1b and the Shaker_S3S4_K v 3.1 chimera, the internal solution contained 115 mM NMG-MES, 2 mM EGTA and 10 mM HEPES adjusted to pH 7.5. Data analysis Details of pulse protocols used to elicit gating or ionic currents were adjusted to determine the biophysical properties of each construct adequately and are shown in the figures or described in legends. The obtained QV and GV curves were fitted with a Boltzmann equation: y =exp(−e z ( V − V 1/2 )/ kT ), where V represents the applied voltage, V 1/2 the midpoint potential at which 50% of the total charge has moved or half of the channels have opened, and z is the valence. Time constants of gating currents Ig ac and Ig deac were determined by fitting the decaying part of the current traces with a single or double exponential function. Ionic Ii ac and Ii deac kinetics were determined by fitting the time-dependent rise in current activation or decay during deactivation with a single or double exponential function, respectively. When a double exponential fit was used, a weighted average time constant was calculated based on the contribution (amplitude) of each component. All results are expressed as mean±s.e.m. with n the number of oocytes analysed. Simulations Simulations were performed in MATLAB using a sequential four-state Markov model of the VSD ( Fig. 7b ). To produce ionic currents, the fourth state was made an open state, and its open probability was used to determine the ionic current based on a reversal potential of −58 mV. Rate parameters at a potential of 0 mV were estimated from K v 3.1b gating and ionic current kinetic data using n = α 0 /( α 0 + β 0 ) and τ 0 =1/( α 0 + β 0 ), where n is the proportion of channels in the final state, α 0 is the rate constant going to that state, β 0 is the rate constant going from that state and τ 0 is the kinetic τ of the experimental state change. For each voltage, rate constants were determined using α = α 0 (exp( z ( V − V 1/2 )/ kT )) and β = β 0 (exp(−z( V − V 1/2 )/ kT )), where V 1/2 =6.2 mV and z p , z l and z s are 3.5, 0.4 and 0.001 respectively, to sum to a total apparent valence of 3.9, as taken from the experimental QV curve for the Kv3.1b channels. How to cite this article: Labro, A. J. et al. K v 3.1 uses a timely resurgent K + current to secure action potential repolarization. Nat. Commun. 6:10173 doi: 10.1038/ncomms10173 (2015).